Perovskite seeding growth of formamidinium-lead-iodide-based perovskites for efficient and stable solar cells Formamidinium-lead-iodide (FAPbI 3 )-based perovskites with bandgap below 1.55 eV are of interest for photovoltaics in view of their close-to-ideal bandgap. Record-performance FAPbI 3 -based solar cells have relied on fabrication via the sequential-deposition method; however, these devices exhibit unstable output under illumination due to the difficulty of incorporating cesium cations (stabilizer) in sequentially deposited films. Here we devise a perovskite seeding method that efficiently incorporates cesium and beneficially modulates perovskite crystallization. First, perovskite seed crystals are embedded in the PbI 2 film. The perovskite seeds serve as cesium sources and act as nuclei to facilitate crystallization during the formation of perovskite. Perovskite films with perovskite seeding growth exhibit a lowered trap density, and the resulting planar solar cells achieve stabilized efficiency of 21.5% with a high open-circuit voltage of 1.13 V and a fill factor that exceeds 80%. The Cs-containing FAPbI 3 -based devices show a striking improvement in operational stability and retain 60% of their initial efficiency after 140 h operation under one sun illumination. Hybrid perovskite solar cells have been developed for efficient solar energy conversion in light of the devices' high power conversion efficiencies (PCEs) and facile processing [1] , [2] , [3] , [4] , [5] , [6] . Processing techniques such as one-step antisolvent crystallization and two-step sequential deposition methods have been developed to produce high-quality perovskite thin films [7] , [8] , [9] , [10] . The perovskite composition is tuned via cation and halide selection to manipulate the bandgap, stability, and transport properties of polycrystalline perovskite films [6] , [11] , [12] , [13] , [14] , [15] , [16] , [17] . Among the broad range of compositions, formamidinium-lead-iodide (FAPbI 3 )-based perovskites with minimal bromide anions and bandgap below 1.55 eV, namely (FAPbI 3 ) 1- x (MAPbBr 3 ) x where x is less than 0.05 (hereafter referred to as FAPbI 3 -based perovskites), are of intense interest for photovoltaic applications: they possess a close-to-ideal bandgap and a certified record PCE of 22.7% [2] , [3] , [10] , [12] , [18] , [19] , [20] , [21] . FAPbI 3 -based perovskite solar cells have demonstrated superior initial performance and dark storage stability; however, the devices exhibit rapid performance degradation following operation at their maximum power point (MPP) even for a few hours under illumination [10] , [19] , [22] , [23] . Their operational stabilty is far inferior to mixed cation-halide perovskites cells with high Bromide content (≥15%) via Cs or Rb incorporation (e.g., Cs-doped (FAPbI 3 ) 0.85 (MAPbBr 3 ) 0.15 and FA 0.83 Cs 0.17 Pb(I 0.83 Br 0.17 ) 3 ) [6] , [14] , [15] , [16] , [17] , [20] , [24] , [25] , [26] , [27] . These studies demonstrate the crucial importance of the Cs cation additive for the long-term photostability of mixed cation-halide perovskites. So far, only via two-step sequential deposition processing have superior-performing FAPbI 3 -based perovskite solar cells been achieved [2] , [3] , [10] , [19] . The lack of Cs cation in the sequentially deposited perovskite films is one important reason for the poor operational stability in previously reported FAPbI 3 -based photovoltaic devices [2] , [3] , [10] , [19] , [20] , [22] . In conventional two-step method, efficient incorporation of Cs in FAPbI 3 -based perovskites is curtailed by the low solubility of inorganic cesium-halide salts (CsX, where X = I, Br, Cl) in alcohols (typically isopropanol, IPA) and the limited diffusion depth of inorganic cations into PbI 2 films [28] . Directly adding CsX in the PbI 2 layer as the first step leads to the formation of the non-perovskite δ-phase CsPbI 3 [29] , [30] , and this leads to a failure to produce efficient photovoltaic devices [22] . In addition to the deficiency of cesium incorporation, perovskite nucleation is poorly controlled in conventional two-step sequential processing: variability in the interdiffusion reaction between PbI 2 and the organic compounds produces a substantial variation in device performance among processing batches [8] , [28] , [31] . To reduce the gap between solar cell efficiency and operational stability, here we devise a perovskite seeding growth (PSG) method that leads to Cs-containing, high-quality FAPbI 3 -based perovskite films with a bandgap below 1.55 eV. This advance enables a significant improvement in device operational stability, device performance, and processing reproducibility of FAPbI 3 -based perovskite solar cells. Inspired by the seed-assisted growth of Si and GaAs semiconductor ingots [32] , [33] , [34] , we incorporate submicron-sized crystalline perovskite seeds in the PbI 2 layer in the two-step sequential deposition. The perovskite seeds act as nuclei for the ensuing perovskite growth when alkylammonium halides react with PbI 2 . We successfully incorporate inorganic cations such as Cs into high-quality perovskite films using Cs-containing perovskite seeds. As a result, we achieve large grain sizes, low trap density, and quasi-single crystallographic orientation in perovskite films via the PSG method. Planar perovskite solar cells processed using the PSG method exhibit a high stabilized PCE of 21.5% and narrow batch-to-batch variation (1.4% absolute PCE). The Cs-containing FAPbI 3 -based perovskite solar cells exhibit a striking improvement in photostability and thermal stability over their non-Cs counterparts and retain over 60% of their initial stabilized efficiency after 140 h operation at MPP under one sun illumination. To the best of our knowledge, this represents the highest operational stability among FAPbI 3 -based perovskite solar cells with bandgaps below 1.55 eV [10] , [19] , [22] , [23] , [35] , [36] , [37] . Fabrication of perovskite thin film via PSG The fabrication of FAPbI 3 -based perovskite films via the PSG method is depicted in Fig. 1a and b . We first prepare a PbI 2 layer that contains submicron-sized perovskite seeds with the composition Cs 0.10 FA 0.78 MA 0.12 PbI 2.55 Br 0.45 (we abbreviate to Cs 0.1 MAFA). Atop the PbI 2 layer, we deposit the mixed organic halide salts FAI/MABr/MACl (0.425/0.065/0.113 M in IPA). As shown in Fig. 1b , the perovskite seeds act as nuclei that facilitate perovskite formation during the diffusion of the organic compounds into the PbI 2 layer. Fig. 1 Perovskite thin films prepared by perovskite seeding growth. a Schematic of fabrication procedure of perovskite films using perovskite seeding growth. b Schematic showing PbI 2 transformation to perovskite starting from perovskite seeds due to the lower energy barrier to perovskite crystallization. c The Gibbs energy G tot as a function of particle radius. G tot consists of a volume term G v and a surface term G s , where γ s and γ v are the surface free energy per unit area and volume free energy per unit volume, respectively; d – e Evolution of G tot during the crystallization process without and with the seed crystal, respectively. In the absence of seed crystal, a nucleus must first be formed, and the nucleus must then overcome the energy barrier G * to grow beyond the critical radius r * (Region I). In the case of perovskite seeds embedded in PbI 2 , the size of the seed crystal is already larger than r * and thus the crystallization commences spontaneously from the seed (Region II) Full size image The kinetics of the crystal growth process can be explained through a Gibbs free energy that includes a volume term ( G v ) and a surface term ( G s ) [8] . Once a new nucleus forms (particle size larger than critical radius r * ), the crystal grows spontaneously during the ensuing reaction process; otherwise, it will disintegrate spontaneously (Fig. 1c ). In the conventional two-step method, the crystallization of perovskites will not occur until the formation of nuclei, for which a critical free energy G * has to be overcome [2] , [3] , [8] , [9] , [10] , [38] as depicted in region I of Fig. 1d . In the PSG method, perovskite growth commences immediately from the perovskite seeds (nucleation centers) when the alkylammonium halide salts are deposited on the PbI 2 film (region II Fig. 1e ). In addition, perovskite seeds facilitate the diffusion and intercalation of organic cations and halide anions into the layered PbI 2 via the PbI 2 /perovskite interface channels [3] , [9] , [39] . This is manifested in a faster perovskite crystallization process along the edges of PbI 2 single crystal (Supplementary Fig. 1 ). To fabricate PbI 2 films containing submicron-sized perovskite seeds, we first prepared two separate solutions of PbI 2 and perovskite precursor. It has been shown that perovskite precursors are dispersed as colloids in processing solvents [40] , [41] , [42] . Following addition of the perovskite precursor colloidal solution into the PbI 2 solution, these colloids are well preserved in the PbI 2 solution, as is evident from their dynamic light scattering and absorption profiles (Fig. 2a and Supplementary Fig. 2 ). A schematic of the solution is given in Fig. 2b . The perovskite seeds are formed in the PbI 2 film by annealing the spin-coated film at 70 °C for 2 min. The formation of crystalline perovskite seeds is confirmed via absorption and photoluminescence (PL) spectra (Fig. 2c–d ). The absorption spectrum of the PbI 2 film with perovskite seeds presents two absorption plateaus at around 520 and 780 nm that originate from PbI 2 and perovskite seeds, respectively [9] . The PL peak position and absorption edge of the PbI 2 film with seeds are the same as that of Cs 0.1 MAFA perovskite seed films processed using the anti-solvent method. The crystalline perovskite seeds fail to form in the PbI 2 film if we directly mix the powder-form precursors within the PbI 2 solution (Supplementary Fig. 3 ). This highlights the importance of solvated colloids of perovskite precursor in the PSG method. Fig. 2 Optical characterization of the PbI 2 film with perovskite seeds. a Dynamic light scattering spectra of the pure PbI 2 solution (0.00028 M), pure perovskite precursor solution (0.00028 M), and the PbI 2 solution mixed with perovskite precursor solution (0.00028 M for PbI 2 and 0.00004 M for perovskite precursor). The size indicates the colloidal particle size in solution. b Illustration of the colloids of perovskite precursor in PbI 2 solution. c , d The absorption and PL spectra of pure PbI 2 film, perovskite seed film with a composition of Cs 0.10 FA 0.78 MA 0.12 PbI 2.55 Br 0.45 , and PbI 2 film with perovskite seeds (seed concentration 14 vol.%). e–f Confocal PL mapping of the intensity ( e ) and peak position ( f ) on the PbI 2 film with perovskite seeds Full size image We applied confocal PL mapping on the sample prepared from PbI 2 solution with 14 vol.% perovskite seeds to obtain the spatial distribution of seeds in the PbI 2 film. Here the seed concentration is defined as the volume fraction of perovskite precursor solution added into the PbI 2 solution. From the PL intensity maps (Fig. 2e ), we see that the perovskite seeds (emissive spots) are well dispersed in the PbI 2 film (non-luminescent background in deep blue). As indicated by the very similar PL peak positions over the mapped region (Fig. 2f ), the perovskite seeds at different locations within the PbI 2 film shall have an almost identical composition. The density of perovskite seeds in the PbI 2 film increases with higher seed concentration in the PbI 2 solution (Supplementary Fig. 4 ). We then carried out in situ PL imaging to investigate the perovskite crystallization process upon the deposition of organic ammonium salts solution onto seed-containing PbI 2 film. We did so by tracking the PL emission evolution of the perovskite phase. Figure 3a (left) shows the PL mapping of the perovskite-seed-PbI 2 solid film before the deposition of the organic ammonium salts. The perovskite crystallization growth starts immediately from the seeds when the ammonium salt solution is placed on the seed-containing PbI 2 film. 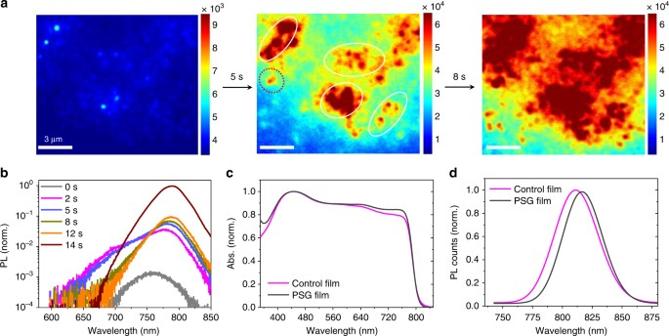Fig. 3 PL imaging of the growth of perovskite seeded films.aIn situ photoluminescence microscopy reports real-time growth of perovskite from the pre-embedded perovskite seeds. The white circles indicate locations with perovskite-seed-assisted growth, while red dashed circles indicate locations with random nucleation process. The color bar indicates the PL intensity emitted from the sample.bThe evolution of PL spectra of a perovskite-seeded region during the reaction process between PbI2and the alkylammonium halides. Note that the substrate was kept at room temperature during the observation.c,dThe absorption and PL spectra of the annealed perovskite films fabricated via conventional two-step sequential deposition (control film) and perovskite seeding growth (PSG film) with 14 vol.% seed concentration. The films were annealed at 140 °C for 25 min. The PL signal was collected from the back side of glass with an excitation wavelength at 540 nm After 2 s, two distinct types of growth kinetics can be observed (Fig. 3a , middle): one is perovskite-seed-assisted growth (white circles) and the other is random nucleation (red dashed circles) without the participation of seeds. The growth rate from the perovskite-seed sites is much faster than growth without the presence of seeds. The growth rate from the perovskite-seed sites reaches about 1 µm s −1 . Overall, the perovskite-seed-assisted growth dominates the perovskite crystallization process across the entire duration of the reaction process (Fig. 3a , right). The time-dependent PL spectra from an area with perovskite seeds show a progressive red-shift in peak position and increased emission intensity with reaction time (Fig. 3b ). This behavior indicates efficient ion exchange between the perovskite seeds and as-formed perovskite crystals during rapid perovskite growth [43] , [44] . We observe a substantially uniform distribution of elements in as-prepared perovskite film after annealing at 140 °C for 25 min, which is evidenced by 2-D element mapping via Time-Of-Flight Secondary Ion Mass Spectrometry (ToF-SIMS) (Supplementary Fig. 5 ). Fig. 3 PL imaging of the growth of perovskite seeded films. a In situ photoluminescence microscopy reports real-time growth of perovskite from the pre-embedded perovskite seeds. The white circles indicate locations with perovskite-seed-assisted growth, while red dashed circles indicate locations with random nucleation process. The color bar indicates the PL intensity emitted from the sample. b The evolution of PL spectra of a perovskite-seeded region during the reaction process between PbI 2 and the alkylammonium halides. Note that the substrate was kept at room temperature during the observation. c , d The absorption and PL spectra of the annealed perovskite films fabricated via conventional two-step sequential deposition (control film) and perovskite seeding growth (PSG film) with 14 vol.% seed concentration. The films were annealed at 140 °C for 25 min. The PL signal was collected from the back side of glass with an excitation wavelength at 540 nm Full size image Characterization of perovskite films Figure 3c and d presents optical characterization of the resulting perovskite films fabricated by the conventional two-step method vs. via the PSG method. We refer to the samples as control and PSG, respectively. Here we observe a similar absorption profile in both control and PSG films (Fig. 3c ). Our FAPbI 3 -based perovskite films achieved here possess a similar absorption edge (815 nm) with previous reports [2] , [3] , [10] . The optical band gap almost remains the same (1.53 eV) for various seed concentrations from 0 to 24 vol.%. From the PL spectra, the full width at half maximum of PL in PSG sample (65 meV) is narrower than that in the control sample (88 meV), indicating reduced energy disorder in the PSG sample (Fig. 3d ). The compositions of control sample and PSG sample (14 vol.% seed concentration) are estimated as (FAPbI 3 ) 0.96 (MAPbBr 3 ) 0.04 and (Cs 0.02 FA 0.98 PbI 3 ) 0.97 (MAPbBr 3 ) 0.03 from the X-ray photoelectron spectroscopy (Supplementary Fig. 6 ), where the Br contents are comparable to previous reports [2] , [3] , [10] . We further explored the chemical depth profiles of different ions in PSG samples via Ar + etching, showing a higher ratio of Br at the top surface than the bottom of samples (Supplementary Fig. 7 ). This leads to different PL peak positions emitted from the surface and bottom of sequentially deposited perovskite film (Supplementary Fig. 8 ). The Cl is negligible in the resulting perovskite films (Supplementary Fig. 7 ), consistent with related previous studies [10] . We next compare the structure and morphology of the perovskite films using X-ray diffraction (XRD) and scanning electron microscopy (SEM). The PSG film has a preferential [001] orientation, while the control film has none as seen from the XRD patterns (Fig. 4a, b ). The preferential orientation in PSG samples may result from that of the seeds in the PbI 2 film that have the lowest interfacial energy. In contrast, there are no (orientable) seeds to modulate perovskite crystallization in the conventional two-step method (Fig. 4a , upper). Fig. 4 Structural and morphological characterization of perovskite films. a XRD patterns of pure PbI 2 film and the as-prepared control perovskite film. The inset is a zoom-in of the XRD spectrum in the range 13°–15°. b XRD patterns of the PbI 2 film with 14 vol.% perovskite seed and the as-prepared PSG perovskite film. The inset is a zoom-in of the XRD spectrum in the range 13 o –15 o . c – d Top-view SEM images of the control and PSG perovskite films. e , f Cross-sectional SEM images of the control and PSG films Full size image The SEM images show that the average grain size (3 µm 2 in lateral area) in the PSG film is much larger than that of the control film (0.25 µm 2 ) (Fig. 4c, d ). We also compare the cross-sections of control and PSG films (around 700-nm thick). The PSG sample clearly shows a columnar character for the crystal grains from the bottom to top (Fig. 4e, f ). The grain size is largely dependent on the nucleation density during the crystallizing process, and it depends as a result on perovskite-seed concentration [4] , [8] . The SEM images and XRD patterns of perovskite films with different seed concentrations are presented in Supplementary Fig. 9 . A seed concentration higher than 14 vol.% leads to more random crystallographic orientation and smaller averaging grain size in the perovskite film. Furthermore, the lattice mismatch between seed and resulting perovskite affects the perovskite growth during the interdiffusion process of the organic compounds. The MAPbBr 3 seed, which has a considerably smaller lattice constant than the target FAPbI 3 -based perovskite, leads to smaller grain size in the resulting perovskite film, and produces lower photovoltaic performance than that of the control sample (Supplementary Fig. 10 ). Photovoltaic devices and performance To evaluate the quality of perovskite films produced by the PSG vs. the conventional two-step sequential method, we fabricated planar solar cells with the device structure ITO/TiO 2 -Cl/perovskite/Spiro-OMeTAD/Au [6] . By plotting the device efficiency vs. seed concentration (Supplementary Fig. 11 ), we observe an obvious increase of efficiency for seed concentrations below 20 vol.% compared to the control devices. We also investigated the effect of seed composition and found that Cs 0.1 MAFA is the best candidate among widely adopted perovskite compositions (Supplementary Fig. 11 ). The highest PCE is achieved for perovskite films fabricated from Cs 0.1 MAFA perovskite seeds with a seed concentration of 14 vol.%. Unless otherwise stated, this optimal condition is used for PSG samples in the text that followings. The histogram of device PCEs for both control and PSG devices is shown in Fig. 5a . The PCE distribution of PSG devices is much narrower than that of control devices, with a significant drop in standard deviation from 3.2 to 1.4% (absolute PCE). The current density-voltage ( J - V ) curves for the best-performing control and PSG devices are shown in Fig. 5b . The open-circuit voltage ( V oc ) of the PSG device increases considerably by 60 mV and the efficiency increases from 19.4 (with V oc = 1.07 V, J sc = 23.7 mA cm −2 , and FF = 0.75) to 21.7% (with V oc = 1.13 V, J sc = 24.1 mA cm −2 , and FF = 0.81) for the reverse scans, where J sc and FF are short-circuit current density and fill factor, respectively. The integrated J sc values from the external quantum efficiency (EQE) spectra are 23.8 and 24.2 mA cm −2 for the control and PSG devices, respectively (Fig. 5c ). 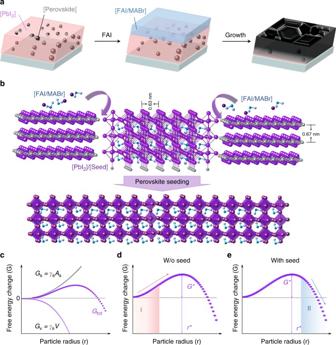The values are consistent with the J sc values determined from J - V curves. Fig. 1 Perovskite thin films prepared by perovskite seeding growth.aSchematic of fabrication procedure of perovskite films using perovskite seeding growth.bSchematic showing PbI2transformation to perovskite starting from perovskite seeds due to the lower energy barrier to perovskite crystallization.cThe Gibbs energyGtotas a function of particle radius.Gtotconsists of a volume termGvand a surface termGs, whereγsandγvare the surface free energy per unit area and volume free energy per unit volume, respectively;d–eEvolution ofGtotduring the crystallization process without and with the seed crystal, respectively. In the absence of seed crystal, a nucleus must first be formed, and the nucleus must then overcome the energy barrierG*to grow beyond the critical radiusr*(Region I). In the case of perovskite seeds embedded in PbI2, the size of the seed crystal is already larger thanr*and thus the crystallization commences spontaneously from the seed (Region II) The hysteresis in best PSG devices is negligible, with a small PCE discrepancy between forward and reverse scans (0.4% absolute PCE), whereas the control device exhibits a considerable hysteresis in J - V scans (Supplementary Table 1 ). The higher degree of hysteresis in control device is mainly due to the higher trap density in the perovskite film as we will discuss later [6] , [45] , [46] . One of our best PSG devices was sent to an accredited PV calibration center (National Institute of Metrology, China) for certification, which confirmed a PCE of 21.9% in reverse scan under AM 1.5G full-sun illumination with a scan rate of 40 mV s −1 (Supplementary Figs. 12 – 13 ). Fig. 5 Photovoltaic performance of control and PSG perovskite solar cells. a Histogram of solar cell efficiencies for control and PSG devices. b J - V curves of the best-performing control and PSG devices with a scanning rate of 10 mV s −1 (voltage step of 10 mV and delay time of 1000 ms) from 1.15 to −0.01 V as the reverse scan, and from −0.01 to 1.15 V as the forward scan. c The external quantum efficiency (EQE) spectra of the control and PSG devices. d Trap density of states obtained by thermal admittance spectroscopy for control and PSG devices Full size image To further investigate the performance improvement by the PSG method, we use thermal admittance spectroscopy to acquire the density of trap states in control and PSG devices [45] , [47] , [48] . The trap density distribution of the control device has two peaks at depth of 0.09 and 0.27 eV, corresponding to trap densities of 0.8 × 10 16 cm −3 and 0.9 × 10 17 cm −3 , respectively. The PSG device shows a strikingly reduced trap density, especially for the deep-level defects. The PSG device shows a reduced trap-mediated recombination rate in impedance spectra (Supplementary Fig. 14 ), and this is accompanied by a longer PL decay lifetime (Supplementary Fig. 15 ) compared to the control device. We also fabricated electron-only and hole-only devices to study the origins of carrier trapping in perovskite films. SCLC reveals that electron traps are dominant in perovskite films (Supplementary Fig. 16 ) [2] , [49] , [50] . The PSG devices exhibit reduced electron traps, in agreement with their higher EQE values in the longer wavelength region as shown in Fig. 5c . 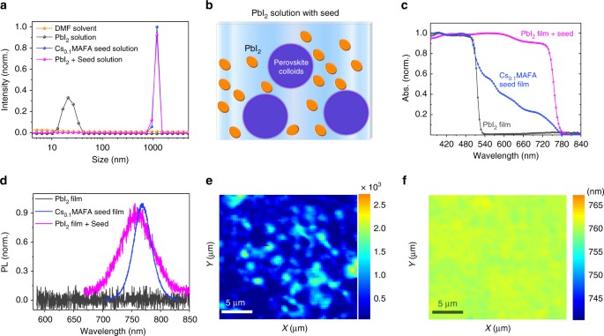Operational stability of perovskite solar cells In addition to the high initial performance, solar cells must have stable output at MPP under constant illumination operating conditions [6] , [15] , [51] . Fig. 2 Optical characterization of the PbI2film with perovskite seeds.aDynamic light scattering spectra of the pure PbI2solution (0.00028 M), pure perovskite precursor solution (0.00028 M), and the PbI2solution mixed with perovskite precursor solution (0.00028 M for PbI2and 0.00004 M for perovskite precursor). The size indicates the colloidal particle size in solution.bIllustration of the colloids of perovskite precursor in PbI2solution.c,dThe absorption and PL spectra of pure PbI2film, perovskite seed film with a composition of Cs0.10FA0.78MA0.12PbI2.55Br0.45, and PbI2film with perovskite seeds (seed concentration 14 vol.%).e–fConfocal PL mapping of the intensity (e) and peak position (f) on the PbI2film with perovskite seeds An addition of a small amount of Cs cations has been previously shown to improve dramatically the photostability and thermal stability of high-performance mixed-cation, mixed-halide perovskite solar cells [6] , [14] , [15] , [16] , [17] , [20] , [36] (Supplementary Table 2 ). As shown in Fig. 6a , in the absence of Cs incorporation (for both control and non-Cs PSG devices), the steady-state output of FAPbI 3 -based perovskite solar cells exhibits an obvious drop in the first 300 s operation under AM1.5 illumination. In contrast, stable output is achieved in the case of the Cs-containing PSG devices. We further examine the long-term operational stability of Cs-containing PSG devices operating at MPP under one sun illumination (Fig. 6b ). These devices were operated at 1 sun MPP for about 10 h, and then stored under dark for about 10 h, and then this cycle was repeated, with the goal of emulating solar cell working conditions [27] , [46] . At the end of each continuous MPP tracking, a reverse-scan efficiency was recorded as well. The device retains 60% of initial stabilized efficiency after 140 h MPP operation (corresponding to 280 h stability test) when direct MPP tracking is employed. It should be noted that there is a discrepancy between steady-state and reverse-scan PCEs after 20 h MPP operation. This highlights the necessity of using MPP tracking, instead of taking the reverse J - V scans for long-term operational stability tests, a point discussed recently by W. Tress et al [27] . Fig. 6 Stability characterization of perovskite solar cells. a The steady-state power output of the control device (w/o Cs) and PSG devices using MAFA (w/o Cs) and Cs 0.1 MAFA (with Cs) seeds measured at MPP under AM 1.5G full-sun illumination. b Long-term operational stability test for the PSG device under AM 1.5G illumination with a 420 nm cutoff UV filter. The device was repeatedly operated at MPP for 10 h, and then stored under dark for 10 h (gray area) under N 2 environment. The reverse-scan efficiency was recorded as well at 100 mV s −1 scan rate after each 10-h MPP operation. The stabilized efficiency at the red point was obtained by replacing the degraded Spiro-OMeTAD layer with a fresh one. c J - V curves of the control device and PSG device before MPP tests and after MPP operation of 300 s for the control device and after MPP operation of 200 h for the PSG device Full size image We further compare the J - V curves of the control and PSG devices before and after degradation (Fig. 6c ). The main efficiency loss in Cs-containing PSG devices after 200-h MPP operation (from 20.7 to 13.8%) and control device after 300-s MPP operation (from 18.7 to 10.9%) originates from losses in J sc and fill factor. The J sc loss in Cs-containing PSG devices arises mainly from deterioration in the Spiro-OMeTAD layer [48] , [52] : when we replace the Spiro-OMeTAD with a fresh layer (Supplementary Fig. 17 ), the J sc value recovers to 23.6 mA cm −2 and the stabilized efficiency recovers to 80% of the initial value (red dot in Fig. 6b ). Thermal stability is another concern in solar applications due to illumination-induced heating. We examine the accelerated thermal decomposition on the perovskite films with and without Cs. The decomposition of perovskite film is strikingly suppressed when Cs-containing perovskite seeds are used (Supplementary Fig. 17 ). In summary, we report a PSG approach to fabricate high-quality, Cs-containing FAPbI 3 -based perovskite films with a bandgap below 1.55 eV. 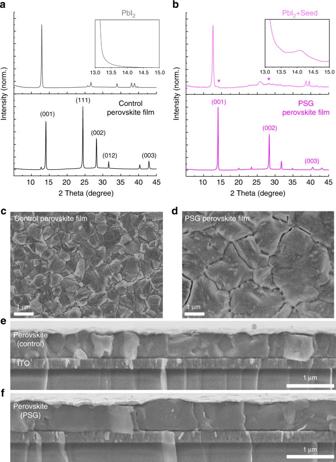Fig. 4 Structural and morphological characterization of perovskite films.aXRD patterns of pure PbI2film and the as-prepared control perovskite film. The inset is a zoom-in of the XRD spectrum in the range 13°–15°.bXRD patterns of the PbI2film with 14 vol.% perovskite seed and the as-prepared PSG perovskite film. The inset is a zoom-in of the XRD spectrum in the range 13o–15o.c–dTop-view SEM images of the control and PSG perovskite films.e,fCross-sectional SEM images of the control and PSG films The perovskite films with seed-assisted growth exhibit large grain size and preferential crystallographic orientation. The perovskites embedded in the PbI 2 film serve as seed crystals that facilitate perovskite growth. Using Cs-containing perovskite seeds, we successfully incorporate Cs cations into FAPbI 3 -based perovskite films. This PSG approach enables us to fabricate high-performance planar perovskite solar cells with significantly enhanced efficiency and operational stability. Further efficiency and stability improvements are expected via advanced defect engineering (e.g., iodide management and interfacial defect passivation) and by using stable hole-transport layer [2] , [19] , [24] . Device fabrication Pre-patterned indium tin oxide (ITO)-coated glass was sequentially cleaned using detergent, acetone, and IPA. TiO 2 -Cl nanocrystal solutions were synthesized based on previous work [6] . The TiO 2 -Cl films (50 nm in thickness) were spin-coated on the ITO substrates at 3000 rpm for 30 s and were then annealed on a hot plate at 150 °C for 30 min in ambient air. The substrates were immediately transferred to the N 2 -filled glovebox after cooling. To make a PbI 2 solution (1.4 M), 760 mg PbI 2 was dissolved in 1 mL DMF and 160 μL DMSO. The clear PbI 2 solution was obtained by stirring at 70 °C for 12 h. For PSG, the perovskite seed solution (1.4 M) was first prepared in 2 mL mixed solvent (DMF/DMSO = 4:1 volume ratio) with different compositions as listed in Supplementary Table 3 . The perovskite seed solution was stirred at 50 °C for 30 min. The PbI 2 /perovskite seed mixed solution was obtained by adding perovskite colloidal solution into the PbI 2 solution. To make FAI/MABr/MACl solution, 1100 mg FAI, 110 mg MABr, and 115 mg MACl were dissolved in 15 mL iso-propanol. The perovskite films were fabricated by two-step sequential deposition. First, the PbI 2 solution or PbI 2 /perovskite seed mixed solution was spin-coated on ITO/TiO 2 -Cl substrates at 1600 rpm for 20 s and 4000 rpm for 50 s. After spin coating, the film was annealed at 70 °C for 2 min. The as-prepared FAI/MABr/MACl solution was subsequently spin-coated on the PbI 2 or PbI 2 /seed layer at 2000 rpm for 20 s. The film was then annealed at 140 °C for 25 min in air with 25% RH. After cooling down to room temperature, the perovskite film was washed again by drop-casting IPA on the surface. The hole-transport layer (Spiro-OMeTAD) was deposited on perovskite films by spin coating a solution (chlorobenzene solvent) containing 65 mg mL −1 Spiro-OMeTAD, 70 μL mL −1 bis(trifluoromethane)sulfonimide lithium salt (170 mg mL −1 in acetonitrile), 20 μL mL −1 tert-butylpyridine, at the rate of 40,000 rpm for 30 s. Spiro-OMeTAD is bought from Xi'an Baolaite Photoelectric Technology Co., Ltd. Finally, 100 nm Au contact was deposited on top of Spiro-OMeTAD by electron-beam evaporation in an Angstrom Engineering deposition system. Solar cell characterization Current density-voltage ( J - V ) curves were obtained by using a Keithley 2400 current-voltage meter under AM1.5G illumination (Newport, Class A). Unless otherwise stated, J - V curves were obtained by using a scanning rate of 100 mV s −1 from 1.15 to −0.01 V with 10 mV voltage step. The steady-state efficiency was measured by setting the bias voltage to the initial V MPP and then tracing the current density. To calculate the photocurrent density, we define the area using an aperture (0.049 cm 2 ) placed on the glass side of device to avoid overestimation of the photocurrent density. EQE measurements were performed using a Newport system (QuantX-300) calibrated by a certified silicon solar cells without any bias light. The stability tests were performed at continuous MPP under AM 1.5G one-sun illumination with a 420 nm long-pass UV-filter under N 2 environment (equivalent to white LED illumination used in other reports). Without filtering the UV illumination from the solar simulator, the efficiency drops faster and irreversibly possibly due to the interface degradation related to TiO 2 (Supplementary Fig. 18 ) [53] , [54] . The cells were purged with nitrogen flow for 1 h in the testing box before MPP tracking to get rid of residual moisture on the surface. The continuous current output was then recorded. No excess encapsulation and preconditioning procedure is used. Optical characterization PL was measured using a Horiba Fluorolog time correlated single-photon-counting system with photomultiplier tube detectors. The light was illuminated from the glass side of the perovskite film. The excitation source is a laser diode at a wavelength of 540 nm. In situ wide-field PL imaging was carried out on a home-built inverted optical microscope (Ti-U, Nikon). An air objective (0.92 NA, 60× magnification) was used. A 488 nm laser line from an argon laser was used as the excitation light. A pair of half-wave and quarter-wave plates were used for converting the linear polarized laser light into the circular-polarized light. A lens was used to expand the laser beam for wide-field excitation. The PL emission collected by the same objective was filtered with a 500 nm long-pass filter before reaching an EMCCD camera (Hamamatsu). The PbI 2 /perovskite film was prepared onto a clean glass cover slide (170 μm in thickness) instead of the thick glass substrate often used for solar cells. FAI/MABr/MACl solution in anhydrous IPA was then dropped on to the film while PL imaging started. PL video was acquired with a frame rate of 50 ms. PL spectral mapping was carried out with 488 nm laser excitation using a home-built confocal microscope on a 20 × 20 μm 2 sample area with a resolution of 100 × 100 pixels. The growth rate of perovskite is obtained by measuring the diameter change of red spot (indicating perovskite) after 5 s reaction. Dynamic light scattering was conducted on DelsaMax PRO light scattering analyzer. A 50 mW diode-pumped solid-state single longitudinal mode laser was used and operated at 532 nm. The DelsaMax Analysis software was used to analyze the light scattering data obtained using the QELS function to determine a hydrodynamic radius. The tube was washed for three times by DMF before injecting the solution. Additional materials characterization High-resolution SEM images were obtained using the Hitachi S-5200 microscope with an accelerating voltage of 1 kV. XRD patterns were collected using a Rigaku MiniFlex 600 diffractometer equipped with a NaI scintillation counter and using monochromatized Copper Kα radiation ( λ = 1.5406 Å). XPS analysis was carried out using the Thermo Scientific K-Alpha XPS system, with a 300 μm spot size, 75 eV pass energy, and energy steps of 0.05 eV. Perovskite thin films were prepared on ITO substrates and electron flood gun was used for charge compensation to avoid peak shifting. All signals were normalized to the Pb signals for direct comparison between different samples. Optical absorption measurements were carried out in a Lambda 950 UV/Vis spectrophotometer. The impedance spectrum was measured using a potentiostat electrochemical workstation (AUT50690, PGSTAT204, The Netherlands) at different biases. The frequency ranges from 1 MHz to 0.01 Hz with 100 data points. The characteristic relaxation time is obtained by using R rec C rec (see equivalent circuit in Fig. S14 ). The Warburg impedance ( W s ) is added to the equivalent circuit due to ion migration in perovskite, which is manifested as a semi-infinite circle at the low-frequency part (below 10 Hz). The defect density is estimated from the frequency-dependent capacitance using the following equation: 
    N_t(f) = - (V_bi - V_app)/qWkT× (dC/df) × f,
 (1) where V bi , W , and V app stand for the build-in voltage, the width of the space charge region, and applied voltage, respectively. The frequency is converted from frequency to energy level of defects ( E a = E t − E c / E v ) using thermal admittance spectroscopy. Then we derived the defect distribution under different bias voltages as a function of energy level: 
    N_t(E_a) = - (V_bi - V_app)/qWkT× (dC/df) × f.
 (2) To identify the energy levels of defects, we adopted used the method to link frequency and energy level in related prior literature [47] . ToF-SIMS measurements were carried out with a time-of-flight secondary ion mass spectrometer (TOF.SIMS 5) from IONTOF company. Ar-ion is used to etch the perovskite layer-by-layer and then the Bi ion is used to create segments with positive or negative charge. The sputtering rate is 0.22 nm s −1 for SiO 2 with 10 KeV energy under GCIB mode. 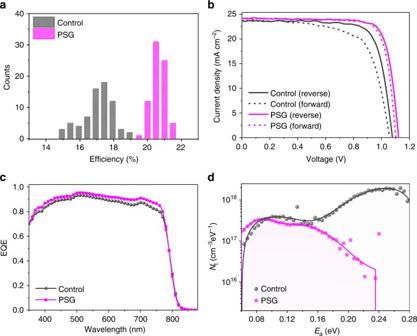Fig. 5 Photovoltaic performance of control and PSG perovskite solar cells.aHistogram of solar cell efficiencies for control and PSG devices.bJ-Vcurves of the best-performing control and PSG devices with a scanning rate of 10 mV s−1(voltage step of 10 mV and delay time of 1000 ms) from 1.15 to −0.01 V as the reverse scan, and from −0.01 to 1.15 V as the forward scan.cThe external quantum efficiency (EQE) spectra of the control and PSG devices.dTrap density of states obtained by thermal admittance spectroscopy for control and PSG devices 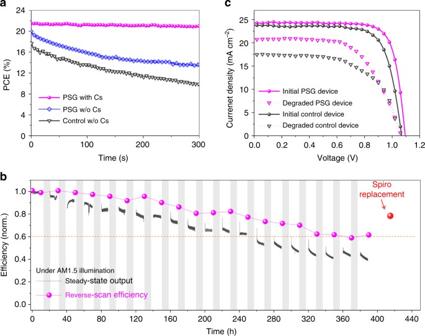Fig. 6 Stability characterization of perovskite solar cells.aThe steady-state power output of the control device (w/o Cs) and PSG devices using MAFA (w/o Cs) and Cs0.1MAFA (with Cs) seeds measured at MPP under AM 1.5G full-sun illumination.bLong-term operational stability test for the PSG device under AM 1.5G illumination with a 420 nm cutoff UV filter. The device was repeatedly operated at MPP for 10 h, and then stored under dark for 10 h (gray area) under N2environment. The reverse-scan efficiency was recorded as well at 100 mV s−1scan rate after each 10-h MPP operation. The stabilized efficiency at the red point was obtained by replacing the degraded Spiro-OMeTAD layer with a fresh one.cJ-Vcurves of the control device and PSG device before MPP tests and after MPP operation of 300 s for the control device and after MPP operation of 200 h for the PSG device The polarity of ionic beam was kept positive. Data availability Data that support the findings of this study are available in separate Supplementary Data Files in Supplementary Information section. All other relevant data are available from the corresponding authors upon reasonable request.